Photo and copper dual catalysis for allene syntheses from propargylic derivatives via one-electron process Different from the traditional two-electron oxidative addition-transmetalation-reductive elimination coupling strategy, visible light has been successfully integrated into transition metal-catalyzed coupling reaction of propargylic alcohol derivatives highly selectively forming allenenitriles: specifically speaking, visible light-mediated Cu-catalyzed cyanation of propargylic oxalates has been realized for the general, efficient, and exclusive syntheses of di-, tri, and tetra-substituted allenenitriles bearing various synthetically versatile functional groups. A set of mechanistic studies, including fluorescence quenching experiments, cyclic voltammetric measurements, radical trapping experiments, control experiments with different photocatalyst, and DFT calculation studies have proven that the current reaction proceeds via visible light-induced redox-neutral reductive quenching radical mechanism, which is a completely different approach as compared to the traditional transition metal-catalyzed two-electron oxidative addition processes. Due to the wide existence of allene unit in natural products, bioactive molecules [1] , and functional materials [2] , development of methods for efficient allene syntheses is of high current interest [3] , [4] , [5] , [6] , [7] , [8] , [9] , [10] , [11] . A few strategies such as allenylic substitution with 2-halo-1,3-butadienes [12] , [13] or allenyl esters [14] , [15] , [16] , [17] , [18] , 1,4-difunctionalization of 1,3-enynes [19] , [20] , [21] , [22] , [23] , [24] , [25] , [26] , [27] , [28] , [29] , [30] , [31] , [32] , allenation of the terminal alkynes (ATA) reaction [33] , [34] , and coupling reactions involving propargylic substrates [35] , [36] , [37] , [38] , [39] , [40] , [41] , [42] , [43] , [44] , [45] , [46] , [47] , [48] , [49] , [50] , [51] , [52] , [53] , have been extensively and well established. For the last reaction, in addition to the S N 2′-type substitution of propargylic substrates [38] , [39] , [40] , [41] , [42] , [43] , [44] , [45] , [46] , transition metal-catalyzed coupling reaction of propargylic alcohol derivatives with organometallic reagents [47] , [48] , [49] , [50] , [51] , [52] , [53] involves a two-electron oxidative addition-transmetalation-reductive elimination process (Fig. 1a ). However, scope and selectivity limitation remain due to the issues of the intrinsic two-electron mechanism [54] , [55] , [56] . Allenenitriles have been frequently employed as useful synthetic precursors for various organic motifs [57] , [58] , [59] , while the classic synthetic method relies on stoichiometric amount of CuCN-mediated cyanation of propargylic alcohols with KCN (1.5 equiv) in the presence of HBr (2.5 equiv) [60] . We envisioned a concept for allenenitrile syntheses via the coupling reaction from propargylic derivatives involving a one-electron process (Fig. 1b ). The challenges here (Fig. 1b ) are (1) the regioselectivity issue on possible formation of alkyne products [61] , [62] , (2) the match of radical reactivity with the transition metal species, and (3) the regeneration of the catalytically transition metal catalyst. Fig. 1: Coupling reactions involving propargylic derivatives. a Traditional transition metal-catalyzed two-electron cross-coupling reactions. b A concept of one-electron process for cross-coupling reactions. c This work: an example of such a concept for allenenitrile synthesis (visible light/transition metal dual catalysis). Full size image In this work, we wish to report such a concept-a radical-based efficient syntheses of allenenitriles from propargylic oxalates and TMSCN under the dual catalysis of photo and copper (Fig. 1c ) [60] . Optimization of reaction conditions We began our study on the coupling reaction of propargylic oxalate 1a with trimethylsilyl cyanide (TMSCN) under blue light irradiation in the presence of CuBr and photocatalyst, fac -Ir(ppy) 3 . 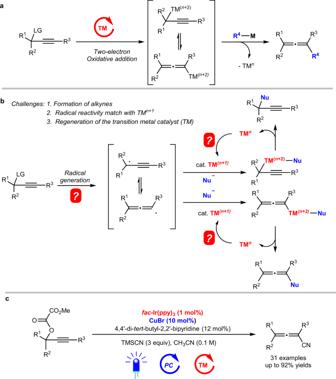Fig. 1: Coupling reactions involving propargylic derivatives. aTraditional transition metal-catalyzed two-electron cross-coupling reactions.bA concept of one-electron process for cross-coupling reactions.cThis work: an example of such a concept for allenenitrile synthesis (visible light/transition metal dual catalysis). The desired allenenitrile 2a was formed in DMF for 24 h in 29% NMR yield with 18% recovery of 1a (Table 1 , entry 1). After evaluation of a series of 2,2′-dipyridine ligands, we were glad to find that 4,4′-di- tert -butyl-2,2′-bipyridine (dtbbpy, L5 ) was the optimal ligand (Table 1 , entries 2–6). Notably, no propargylic isomer 3a was detected in the crude reaction mixture. The reaction performed in CH 3 CN gave higher yield than other checked solvents such as DMAC, NMP, DMPU, THF, and DCM (Table 1 , entry 7, for details on solvent screening, see the Supplementary Information ). Increasing the loading of TMSCN (Table 1 , entry 8) and running the reaction at a concentration of 0.1 M (Table 1 , entry 9) further promoted the formation of 2a , which could be isolated in 89% yield on a 0.5 mmol reaction scale. As expected, CuBr 2 was totally ineffective (Table 1 , entry 10). No reaction occurred in the absence of the light (Table 1 , entries 11 and 12) or photocatalyst fac -Ir(ppy) 3 (Table 1 , entry 13), suggesting that both the light and photocatalyst were indispensable for the transformation. Table 1 Optimization of the reaction conditions. Full size table Substrate scope With the optimized reaction conditions in hand, we set out to investigate the substrate scope of this method (Fig. 2 ). Overall, a variety of terminal tertiary propargylic oxalates smoothly underwent cyanation to form trisubstituted allenenitriles as exclusive regioisomer in good to excellent yields. No obvious yield difference among cyclic ( 2a , 2b , 2c , 2d ) and acyclic ( 2i , 2j , 2m ) substrates was observed. Even with the sterically hindered adamantyl-containing oxalate 1l , the yield of 2l was 91% after increasing the catalyst loadings of CuBr and L5 to 15 mol% and 18 mol%, respectively. A wide range of reactive yet synthetic useful functional groups, such as sulfide ( 2e , easily poisoning Cu catalysis), amide ( 2f ), halogen ( 2n , 2o , 2p ), ester ( 2k , 2q ), ketal ( 2g , 2s ), terminal alkyne ( 2q ), and terminal olefin ( 2r ) were intact under the standard mild reaction conditions. Interestingly, under the standard conditions the propargylic oxalate 1h with a ketone unit was converted to nitrile 2h with the in situ formation of a synthetically useful enol silyl ether entity [63] , [64] in 65% yield. The thiophene unit in substrate 1t was also accommodated. Furthermore, products incorporating Boc-protected L-proline 2u , pentoxyifylline 2v , Boc-protected tropinone 2w and 2w’ , and raspberry ketone tetra- O -acetyl-β-D-glucopyranoside 2x , mestranol 2y worked well without affecting the other fragile functionalities. The structure of 2w’ was unambiguously established by its X-ray analysis. The reaction could be easily conducted on gram-scales ( 2q and 2y ), demonstrating the practicality of this protocol. Even the reaction of terminal secondary propargylic oxalates 1z and 1A still afforded 1,3-disubstituted allenenitriles 2z and 2A as the products in decent yields and a very high allene/alkyne selectivity (25:1 and 14:1). 4-Phenylallenenitrile 2J could also be obtained via the current method in 54% yield as the only isomer, and the slightlylower isolated yield may be attributed to its instability. Fig. 2: Substrate scope study. a CuBr (15 mol%) and L5 (18 mol%) were used. b Due to the difficulty of separating the two regioisomers, the yield value refers to the isolated yield of a mixture of alkyne and allene; the regioselectivity was determined by 1 H NMR analysis. c The reaction was conducted in 10 mL CH 3 CN. Full size image The reaction could be further extended to non-terminal propargylic oxalates, such as 1B , 1C , and 1K . When trimethylsilyl-substituted alkyne 1C was used, TMS-substituted allenenitrile 2C was produced exclusively in 88% yield, which was not readily accessible by other ways [65] and very useful in propargylation reaction [66] , [67] . For non-terminal propargylic oxalates with R 3 being Ph ( 1D ) and CO 2 Me ( 1E ), dinitrile products 4a and 4b were obtained, which must be produced from the subsequent conjugate addition of TMSCN with the in situ formed allenenitrile intermediate 2D and 2E , respectively. Interestingly, when MgCl 2 or MgBr 2 •6H 2 O replaced TMSCN as the nucleophile, various chloroallene or bromoallene bearing sterically hindered adamantyl ( 12l or 13l ), ketal ( 12s ), ester, or terminal alkyne ( 13q ) could be obtained in decent yields. As a comparison, TMSBr or TMSCl gave inferior results (Fig. 3 ). Fig. 3: Reaction with MgCl 2 or MgBr 2 •6H 2 O instead of TMSCN. The reaction condition A was used for the synthesize of cholorallenes (present in red color), and the reaction condition B was used for the synthesize of bromoallenes (present in blue color). Full size image Synthetic applications These allenenitriles are synthetic versatile as shown in Fig. 4 : The Cu(I) catalyzed [4 + 2] cycloaddition [68] of 2a (R 1 , R 2 = -(CH 2 ) 5 -) with furan provided 7-oxa-bicyclo-[2.2.1]heptene derivatives endo - 5 and exo - 5 in 55 and 14% yield, respectively. The configuration of endo - 5 was unambiguously identified by X-ray analysis. Conjugate addition of 4-methylbenzenethiol with 2a afforded sulfur-substituted tetrasubstituted alkene 6 in an excellent yield [69] . Deuteration of α-H of 2m (R 1 = Me, R 2 = -(CH 2 ) 2 Ph) with D 2 O in the presence of K 2 CO 3 and n -Bu 4 NBr readily yielded d - 2m in 96% yield with 96% D-incorporation. Hydrolysis of nitrile group in 2l (R 1 = Me, R 2 = 1-adamantyl) with a base produced allenyl amide 7 in 64% yield [70] . In addition, the ethynyl group in 2q underwent the Cu-catalyzed click reaction with anti-HIV drug AZT (Zidovudine) [71] while the allenenitrile unit remained unreacted, offering useful handle for further synthetic elaboration. Fig. 4: Synthetic transformations of allenenitriles. Reagents and conditions: (a) 2a (0.2 mmol), Cu(CH 3 CN) 4 BF 4 (20 mol%), freshly distilled furan (2 mL), 50 °C, 2 d; (b) 2a (0.4 mmol), 4-methylbenzenethiol (1.2 equiv), Et 3 N (2.0 equiv), CHCl 3 , rt, 24 h; (c) 2 m (0.27 mmol), K 2 CO 3 (5.0 equiv), n -Bu 4 NBr (1.0 equiv), Toluene/D 2 O = 9:11, rt, 2.5 d; (d) 2 l (0.2 mmol), NaOH (20 mol%), Na 2 CO 3 (1.0 equiv), H 2 O 2 (3.9 equiv), EtOH/H 2 O = 5:1, rt, 24 h; (e) 2q (0.4 mmol), AZT (1.0 equiv), CuSO 4 ·5H 2 O (5 mol%), sodium ascorbate (15 mol%), DCM/H 2 O = 1:1. Full size image Mechanistic studies To probe the reaction mechanism, we conducted a set of mechanistic studies. First, several propargylic compounds with different leaving groups 1F (Boc), 1G (Ac), 1H (CO 2 Me) were prepared. The Cyclic Voltammetry (CV) experiments were performed to measure the reduction potential of these substrates 1d , 1F , 1G , and 1H (Fig. 5a ). The half peak potential of redox active oxalate 1d was determined to be E p/2 [ 1d / 1d •- ] = −1.71 V vs SCE (Saturated calomel electrode) in CH 3 CN. However, under the same measurement conditions for 1F (Boc), 1G (Ac), and 1H (CO 2 Me), no apparent anodic and cathodic current peaks could be observed in the range of −3.0 to 0 V, suggesting that these were redox-inactive leaving groups. Indeed, when 1F (Boc), 1G (Ac), or 1H (CO 2 Me) were subjected to the optimal conditions, 100% of the corresponding unreacted starting materials were recovered. Fig. 5: Mechanistic studies. a Experiments and cyclic voltammograms of different propargylic compounds. b Stern-Volmer quenching experiments of fac -Ir(ppy) 3 . c Reaction with Ph-PTZ photocatalyst. d The radical trapping experiment with TEMPO. e Reaction with Ir(dtbbpy)(ppy) 2 PF 6 or Ir[dF(CF 3 )ppy] 2 (dtbbpy)PF 6 as photocatalyst. Full size image Two possible reaction pathways for this transformation based on CV data were proposed as shown in Fig. 6a and Supplementary Fig. 5 . In oxidative quenching cycle (Supplementary Fig. 5 ), first, the excited state of fac -Ir(ppy) 3 * ( E 1/2 red [Ir IV /Ir III* ] = −1.73 V vs SCE in CH 3 CN) [72] could be quenched with oxalate 1 ( E p/2 [ 1d / 1d •- ] = −1.71 V vs SCE in CH 3 CN) to generate [ fac -Ir(ppy) 3 ] + species and anionic radical intermediate 9 , which would form propargylic radical 10 by releasing oxalate anion. Then LCu I CN ( E p/2 red [Cu II /Cu I ] = +0.15 V vs SCE in CH 3 CN, see Supplementary Information for details) would be oxidized by [ fac -Ir(ppy) 3 ] + ( E 1/2 red [Ir IV /Ir III ] = +0.77 V vs SCE in CH 3 CN) [72] to produce LCu II CN, which would further react with TMSCN to yield LCu II (CN) 2 . 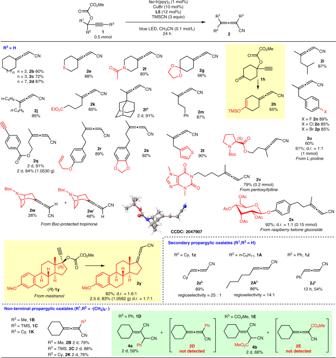Fig. 2: Substrate scope study. aCuBr (15 mol%) andL5(18 mol%) were used.bDue to the difficulty of separating the two regioisomers, the yield value refers to the isolated yield of a mixture of alkyne and allene; the regioselectivity was determined by1H NMR analysis.cThe reaction was conducted in 10 mL CH3CN. Alternatively, in reductive quenching cycle (Fig. 6a ), the excited state of fac -Ir(ppy) 3 * ( E 1/2 red [Ir III* /Ir II ] = +0.31 V vs SCE in CH 3 CN) [72] could be quenched with LCu I CN to generate LCu II (CN) and [ fac -Ir(ppy) 3 ] − species ( E 1/2 red [Ir III /Ir II ] = −2.19 V vs SCE in CH 3 CN) [72] . Oxalate 1 could be reduced by [ fac -Ir(ppy) 3 ] − to yield anionic radial intermediate 9 via one-electron reduction. Finally, in both pathway the radical intermediate 10 may isomerize to allenyl radical 11 [73] , [74] , which may bind with LCu II (CN) 2 , followed by reductive elimination to deliver allenenitrile 2 and regenerate the catalytically active species LCu I CN. Another possible pathway, 11 could abstract the CN group from LCu II (CN) 2 to afford allenenitrile 2 [32] , [75] , [76] . The steric effect of R 1 , R 2 , and R 3 may play an important role in the reaction selectivity for forming 2 or 3 . Fig. 6: Possible mechanism. 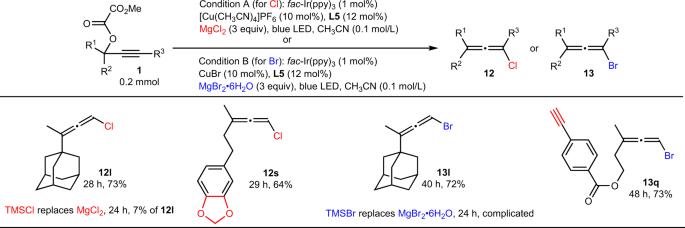Fig. 3: Reaction with MgCl2or MgBr2•6H2O instead of TMSCN. The reaction condition A was used for the synthesize of cholorallenes (present in red color), and the reaction condition B was used for the synthesize of bromoallenes (present in blue color). a Proposed mechanism via reductive quenching cycle. b Free energy profiles calculated for the reaction of L4 Cu II (CN) 2 with Int1 . Relative free energies are given in kcal/mol. Full size image To distinguish the two pathways, Stern-Volmer quenching experiments of fac -Ir(ppy) 3 were carried out. As shown in Fig. 5b , the excited state of the photocatalyst fac -Ir(ppy) 3 was efficiently quenched by the CuBr/ L5 catalyst. Furthermore, if the cyanation of 1d would be realized via oxidative quenching cycle, considering the redox-potential window of typical photocatalysis (Ir/Ru/organic-PC etc.) [77] , the Ph-PTZ was selected as another potential photocatalyst for this transformation. The reaction in the presence of photocatalyst Ph-PTZ instead of fac -Ir(ppy) 3 would provide readily radical 10 or 11 , the subsequent SET process between the oxidized state of Ph-PTZ + ( E 1/2 [Ph-PTZ + /Ph-PTZ] = +0.815 V vs SCE in CH 3 CN) [61] and LCu I CN ( E p/2 red [Cu II /Cu I ] = +0.15 V vs SCE in CH 3 CN) would form LCu II CN, which could yield 2d . However, such a reaction only afforded 10% of 2d with 90% of 1d being recovered (Fig. 5c ). When 2 equiv of TEMPO were used as the radical trapping agent in the reaction of 1d , the formation of 2d was obviously reduced (16% vs 87%), and the TEMPO-trapped product 14 and/or 15 could be detected by LC-HRMS analysis, which supports the involvement of radical intermediates in the current transformation (Fig. 5d ). Furthermore, in order to check the possible triplet energy transfer mechanism, other ruthenium- or iridium-based dyes or organic photocatalysts were tested under standard conditions (for details on photocatalyst screening, see the Supplementary Information ): Photocatalysts (Ir(dtbbpy)(ppy) 2 PF 6 , E T = 49.2 kcal/mol and Ir[dF(CF 3 )ppy] 2 (dtbbpy)PF 6 , E T = 60.8 kcal/mol) with its triplet energy similar to that of fac -Ir(ppy) 3 ( E T = 57.8 kcal/mol) did not provide 2d at all (Fig. 5e ) [78] , [79] . To further elucidate the reaction mechanism, density functional theory (DFT) calculations were preformed to survey the reaction of 1B using ligand L4 (For details on DFT calculations, see the Supplementary Information and Supplementary Data 1 ). As proposed by Fig. 6a , radical intermediate Int1 could be formed from oxalate 1B . Mulliken atomic spin density analysis of Int1 suggests that the single electron distributes on C 1 and C 2 with a similar spin density (0.64 and 0.47, Fig. 6b ), indicating Int1 is a combination of resonance forms of allenyl radical and propargylic radical. As an allenyl radical, Int1 reacts with L4 Cu II (CN) 2 via a singlet diradical transition structure TS1_a with a free energy barrier of 10.1 kcal/mol, providing a closed-shell propargyl-Cu(III) complex Int2_a reversibly. Subsequent reductive elimination produces the final allenenitrile product 2B with a very low barrier of 1.0 kcal/mol ( TS2_a ). Furthermore, the concerted radical cyanation process is also investigated. 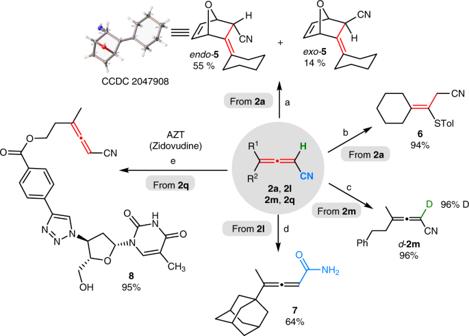Fig. 4: Synthetic transformations of allenenitriles. Reagents and conditions: (a)2a(0.2 mmol), Cu(CH3CN)4BF4(20 mol%), freshly distilled furan (2 mL), 50 °C, 2 d; (b)2a(0.4 mmol), 4-methylbenzenethiol (1.2 equiv), Et3N (2.0 equiv), CHCl3, rt, 24 h; (c)2m(0.27 mmol), K2CO3(5.0 equiv),n-Bu4NBr (1.0 equiv), Toluene/D2O = 9:11, rt, 2.5 d; (d)2l(0.2 mmol), NaOH (20 mol%), Na2CO3(1.0 equiv), H2O2(3.9 equiv), EtOH/H2O = 5:1, rt, 24 h; (e)2q(0.4 mmol), AZT (1.0 equiv), CuSO4·5H2O (5 mol%), sodium ascorbate (15 mol%), DCM/H2O = 1:1. A triplet transition structure TS_a was obtained with a much higher free energy barrier of 30.3 kcal/mol, which indicates that the stepwise pathway via a Cu(III) intermediate is more favorable. On the other hand, the possibility of Int1 acting as a propargyl radical has also been considered. A similar oxidation/reductive elimination process is obtained, but more energy demanding, due to the steric effect caused by the cyclohexyl group with the ligand. Thus, allenenitriles 2B were generated as the only products. 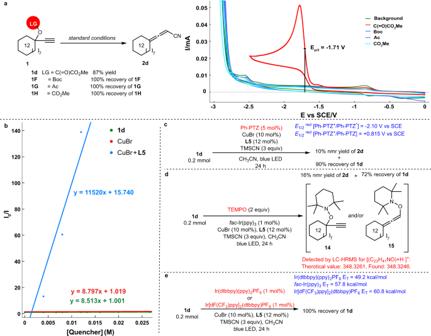Fig. 5: Mechanistic studies. aExperiments and cyclic voltammograms of different propargylic compounds.bStern-Volmer quenching experiments offac-Ir(ppy)3.cReaction with Ph-PTZ photocatalyst.dThe radical trapping experiment with TEMPO.eReaction with Ir(dtbbpy)(ppy)2PF6or Ir[dF(CF3)ppy]2(dtbbpy)PF6as photocatalyst. 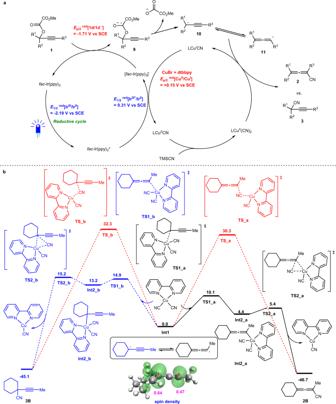Fig. 6: Possible mechanism. aProposed mechanism via reductive quenching cycle.bFree energy profiles calculated for the reaction ofL4CuII(CN)2withInt1. Relative free energies are given in kcal/mol. These above results definitely confirmed that the reductive quenching cycle in Fig. 6a was the dominant pathway in the current transformation, which is different from the well-established oxidative quenching mechanism [61] , [75] , [76] . In conclusion, we have developed a general and efficient method for the highly selective synthesis of di-, tri-, and tetra-substituted allenenitriles from readily available propargylic oxalates and TMSCN under photoredox conditions. This reaction featured mild conditions and a broad functional group compatibility. Excellent regioselectivities were achieved in both terminal and internal propargylic oxalates. Even for secondary substrates, allenenitriles were still the predominant products. The current method was further extended to the synthesis of cholorallenes or bromoallenes by using MgCl 2 or MgBr 2 •6H 2 O as the nucleophile. Stern-Volmer quenching experiments, cyclic voltammetric measurements, radical trapping experiments, control experiments with different photocatalysts, and DFT calculation studies indicated that propargylic radical and allenyl radical generated via light-induced one-electron process were involved via the reductive quenching cycle. This protocol for allenenitrile syntheses involving one-electron mechanistic pathway is very different from the traditional transition metal-catalyzed two-electron coupling reactions and will surely overcome the scope limitation of the known protocols and enjoy scopes for the efficient syntheses of differently functionalized allenes due to the powerful catalytic activity of copper [80] , [81] . Further studies on highly selective allene synthesis via such one-electron process and other photocatalysts are being actively pursued in this laboratory. General procedure for the copper-catalyzed cyanation of propargylic oxalates To a flame-dried 10 mL Schlenk tube were added fac -Ir(ppy) 3 (3.3 mg, 5 μmol), CuBr (7.3 mg, 0.05 mmol), 4,4′-di- tert -butyl-2,2′-bipyridine L5 (16.4 mg, 0.06 mmol), 1a (105.4 mg, 0.5 mmol)/CH 3 CN(2.5 mL), and TMSCN (157.2 mg, 1.5 mmol)/CH 3 CN(2.5 mL) sequentially under Ar atmosphere. The resulting mixture was irradiated with a 50 W blue LED lamp (2-3 cm away, with cooling fan to keep the reaction temperature at 35–40 °C) for 24 h with stirring and monitored by TLC. The resulting mixture was filtrated through a short pad of silica gel eluted with ethyl ether (30 mL). After evaporation, the residue was purified by chromatography on silica gel to afford the pure product 2a .